Vertical atomic manipulation with dynamic atomic-force microscopy without tip change via a multi-step mechanism Manipulation is the most exciting feature of the non-contact atomic force microscopy technique as it allows building nanostructures on surfaces. Usually vertical manipulations are accompanied by an abrupt tip modification leading to a change of contrast. Here we report on low-temperature experiments demonstrating vertical manipulations of ‘super’-Cu atoms on the p (2 × 1) Cu(110):O surface, both extractions to and depositions from the tip, when the imaging contrast remains the same. These results are rationalized employing a novel and completely general method that combines density functional theory calculations for obtaining energy barriers as a function of tip height and a Kinetic Monte Carlo algorithm for studying the tip dynamics and extraction of manipulation statistics. The model reveals a novel multi-step manipulation mechanism combining activated jumps of ‘super’-Cu atoms to/from the tip with their drag by and diffusion on the tip. The ability of scanning probe microscopies, such as scanning tunnelling microscopy (STM) and non-contact atomic force microscopy (NC-AFM), to scan surfaces with atomic/molecular resolution [1] and provide in some cases information on the chemical identity of the scanned atoms [2] , has placed these methods at the top of the list of the experimental toolkit of surface science. However, the most exciting applications of either of the techniques are related to their ability to perform nano-manipulation [3] , [4] , [5] . Both lateral [6] , [7] , [8] and vertical [9] , [10] , [11] manipulations have been used to build bottom-up nanostructures on surfaces. The latter manipulation, where the manipulated atom is either dropped to or extracted from the surface, normally results in a modification of the tip apex with the concomitant change of the image contrast. Compared to STM, the NC-AFM technique is more versatile, since the force between tip and surface is effectively measured, and therefore this method can be applied to surface imaging and manipulation of any material. In all cases of both vertical and lateral NC-AFM manipulations at room temperature reported so far, it was assumed that the species are displaced thermally in a single elementary event triggered simply by the reduction of relevant energy barriers. The barriers are lowered due to tip proximity as compared with the situation of the tip being sufficiently far away from the species when the barrier is large, making the species essentially immobile. In comparison with STM, a unique advantage of NC-AFM in nano-manipulation is concerned with the fact that the tip oscillates and hence the energy barriers are periodically modified. This unique feature allows accessing processes that in microscopes operating at fixed tip–sample distance, such as STM, would be inaccessible. A characteristic signature of a successful manipulation event using NC-AFM is an incomplete image of the surface object being manipulated. For instance, if an atom is picked up vertically by the tip during the scan, only the initial part of a circular blob representing the atom is imaged, the rest is missing and the image is terminated by a straight line running along the fast imaging direction (a ‘half-moon’ image). In the opposite case of an atom being deposited from the tip to the surface, the final part of the circular blob shows up starting with a straight line along the fast imaging direction [12] . In fact, in most cases reported so far after such a vertical manipulation the whole contrast abruptly changes [12] as the tip apex structure changes significantly after the manipulation event. Note that in the case of the lateral manipulation there are two spots of the manipulated atom on the same image: the first one shows the atom’s initial position and is terminated abruptly (a ‘half moon’), while the second one corresponds to the atom’s new position. For a lateral manipulation it is natural to assume that the tip structure remains the same before and after the manipulation event, and this fact enables, at least in principle, collecting the corresponding statistics. The situation is not that simple in the case of the vertical manipulation, as the tip apex structure is bound to change, making accumulation of reliable statistical information difficult. Therefore, understanding vertical manipulation mechanisms poses a real challenge for both experiment and theory. Here we report on a joined experimental and theoretical study of low-temperature NC-AFM experiments of vertical manipulations of ‘super’-Cu atoms on the p (2 × 1) phase of oxidized Cu(110) surface, both extractions to and depositions from the tip, which leave the imaging contrast unchanged after each manipulation event. To rationalize these observations we have developed a new and completely general theory applicable to both vertical and lateral manipulations that takes explicit account of the tip movement in NC-AFM. The model reveals a novel multi-step manipulation mechanism combining activated jumps of ‘super’-Cu atoms to/from the tip with their drag by and diffusion on the tip. We note that copper surfaces are important in their own right as industrial catalysts [13] , and surface oxidation is believed to play a crucial role in their catalytic activity [14] . Summary of main results The results of vertical NC-AFM manipulation of ‘super’-Cu atoms on the p (2 × 1) Cu(110):O surface are shown in Fig. 1 . Both depositions and extractions of atoms to/from the surface have experimentally been performed and theoretically analysed in unprecedented detail. The experimental system and our theoretical analysis exhibit a few unique features: (1) the contrast before and after the vertical manipulation events remains essentially the same, that is, the tip apex structure must be changing only in its secondary features; (2) extensive theoretical modelling leads to an explanation of the mentioned contrast stability in terms of a multi-step model, involving unexpected processes at the apex after picking up/disposing of an atom; (3) kinetic simulations based on a Kinetic Monte Carlo (KMC) algorithm [15] were performed to include the tip motion, slow at atomic time scale, and to provide access to the realistic calculations of the likelihood of the extraction and deposition manipulations. 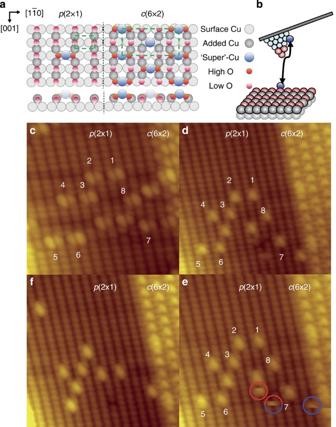Figure 1: NC-AFM imaging and manipulation. (a) Ball model (top and side views) of thep(2 × 1) phase (on the left) immediately next to thec(6 × 2) phase (on the right) with unit cells of 5.10 × 3.61 and 15.30 × 7.22 Å2, respectively, shown by a green dashed line. Note that at intermediate oxygen exposures, when both phases are formed next to each other, Cu atoms adsorb also on thep(2 × 1) surface as adatoms in geometries very similar to those of the ‘super’-Cu atoms of thec(6 × 2) surface (one such atom is shown on the left). (b) Schematic model of vertical manipulations leaving the tip apex chemical identity unchanged. (c–f) The same area of the surface as imaged by (c) Cu- and (d–f) O-terminated tips. Slow scan direction is vertically down. For ease of comparison, spots corresponding to the same super-Cu atoms are numbered identically inc–e. Notice that the same contrast is found on thec(6 × 2) island and thep(2 × 1) terrace for the super-Cu atoms inc,d: these are observed either as double (c) or as single (d) spots. Images (d–f) were taken during the same experimental run but not necessarily immediately one after the other. One can clearly see a number of vertical manipulations on thep(2 × 1) terrace corresponding to extractions (blue circles) and depositions (red circles) of the Cu adatoms during imaging. Figure 1: NC-AFM imaging and manipulation. ( a ) Ball model (top and side views) of the p (2 × 1) phase (on the left) immediately next to the c (6 × 2) phase (on the right) with unit cells of 5.10 × 3.61 and 15.30 × 7.22 Å 2 , respectively, shown by a green dashed line. Note that at intermediate oxygen exposures, when both phases are formed next to each other, Cu atoms adsorb also on the p (2 × 1) surface as adatoms in geometries very similar to those of the ‘super’-Cu atoms of the c (6 × 2) surface (one such atom is shown on the left). ( b ) Schematic model of vertical manipulations leaving the tip apex chemical identity unchanged. ( c – f ) The same area of the surface as imaged by ( c ) Cu- and ( d – f ) O-terminated tips. Slow scan direction is vertically down. For ease of comparison, spots corresponding to the same super-Cu atoms are numbered identically in c – e . Notice that the same contrast is found on the c (6 × 2) island and the p (2 × 1) terrace for the super-Cu atoms in c , d : these are observed either as double ( c ) or as single ( d ) spots. Images ( d – f ) were taken during the same experimental run but not necessarily immediately one after the other. One can clearly see a number of vertical manipulations on the p (2 × 1) terrace corresponding to extractions (blue circles) and depositions (red circles) of the Cu adatoms during imaging. Full size image The surface systems At the experimental oxygen exposures the oxidized Cu(110) surface consists of p (2 × 1) and c (6 × 2) patches [12] , [16] . The p (2 × 1) surface shown in Fig. 1a on the left has an alternating row/missing row conformation [17] , [18] in the direction, where along the [001] rows alternating Cu and O atoms lie. Occasionally additional Cu adatoms are found on the p (2 × 1) patches on the surface as well, which are bonded between two oxygen atoms as shown in the left part of the figure. Note that a periodic arrangement of such adatoms on a slightly different Cu–O row structure constitutes the c (6 × 2) reconstruction of this surface shown in the right part in Fig. 1a . The additional Cu atoms lie higher than all other surface atoms and have thus acquired the name ‘super Cu atoms’ [17] , [18] , and the two O atoms on either side of them are raised slightly out of plane and move closer to their super Cu, acquiring the names ‘high’ [17] or ‘buckled’ [18] O atoms. Tip preparation During the course of the experiment, we were able, using the method of ref. 12 , to interchange the chemical identity of the tip between O- and Cu-terminated. Two types of NC-AFM images were routinely obtained, shown in Fig. 1c–f , where a p (2 × 1) patch (seen on the left) is positioned next to a c (6 × 2) reconstructed island (on the right): (i) in (c) rows of single bright spots are seen in the p (2 × 1) patch, while double spots appear at the positions of high O atoms around ‘super’-Cu atoms on the c (6 × 2) patch, and (ii) shown in (d) are single spots that are seen for both patches. Although the chemical identity of the rows of bright spots on the p (2 × 1) surface cannot be identified from the images of this phase alone [16] , this, as well as the chemical identity of the tip apex atom, can unequivocally be identified from the image of the c (6 × 2) surface [12] : ‘super’-Cu atoms are imaged with the O-terminated tips and appear as single bright spots, while high-O atoms are imaged with the Cu-terminated tips and appear as double bright spot features. Therefore, by inspecting the contrast in the image of the c (6 × 2) island, we can identify the Cu-terminated tip in (c) and O-terminated tip in (d). In the following, only images like (d–f) related to the O-terminated tip will be considered. NC-AFM vertical manipulation of ‘super’-Cu atoms A typical sequence of three NC-AFM images of the surface taken during the same experimental run (in chronological order but not necessarily one after the other) with an O-terminated tip is shown in Fig. 1d–f . This incidentally means that Cu atoms are imaged on the p (2 × 1) terrace in these images by this tip. In all images we can also see bright spots in the middle of the p (2 × 1) terrace, some of which are numbered for ease of comparison. The identity of the spots in the images can be identified as adsorbed Cu atoms. Indeed, these are single spots in images (d–f) taken with an O-terminated tip; the spots are positioned exactly between two Cu–O rows and exactly between four Cu atoms in these rows (recall that only Cu atoms are imaged in these rows), that is, it must be between two O atoms as shown on the left side of the ball model in Fig. 1a . At the same time, the same location on the surface appears in image (c) as double features (compare the numbered spots in images (c) and (d)): since image (c) must have been taken with the Cu-terminated tip, the observed bright features should be related to the shifted high O atoms on both sides of the ‘super’-Cu adatoms. This amazing similarity in how separate species on the two reconstructions are imaged with both tip terminations confirms our assignment for the additional spots imaged on the p (2 × 1) terrace to correspond to ‘super’-Cu atoms as in the ball model in Fig. 1a . As shown below, our density functional theory (DFT) calculations confirm this model; they also show that the ‘super’-Cu atoms have a very similar structure in both surface phases. Let us now compare images (d) and (e) of Fig. 1 . Several elementary manipulation events take place: two additional spots (two Cu atoms) appear in (e) on the left of the spot numbered 7. One of the spots in (e) has an abrupt termination on the upper side, which is a signature of a deposition of an atom after image (d) was taken. The other feature in (e) corresponds to an atom that was initially deposited and then, after some time during the same scan, extracted (since this spot has abrupt terminations both at the top and at the bottom), and the forthcoming image (not shown) confirms that. In addition, we see another Cu atom in (e) with abrupt termination in the lower part and hence corresponding to a Cu atom extracted during the scan. Similar events are seen in many other images we took in this and similar experimental runs showing multiple atom depositions and extractions, see Supplementary Information . The fact that we have been able to perform these manipulations in a systematic and controlled way, so that a definite outcome was obtained after a certain number of oscillation cycles related to the corresponding probabilities (to be discussed below), is documented in (f), where the letter ‘X’ was written on the p (2 × 1) terrace by a sequence of deposition/extraction manipulations. What we find the most surprising in all these images was that the contrast during these multiple vertical manipulation events remains the same, that is, Cu atoms are interchanged between the tip and surface multiple number of times; however, the chemical identity of the tip apex atom does not change at all and still stays as an O atom. This can only signify that when a Cu atom is picked up from the surface it must be diffusing up the tip structure away from the apex, see the cartoon in Fig. 1b ; conversely, it diffuses down and gets adsorbed on the surface in a ‘super’-Cu position during vertical manipulation events corresponding to depositions. We also find that experimentally the deposition events were easy to perform, while extraction manipulations were very rare. Unfortunately, due to the nature of these manipulations, we found it difficult to experimentally quantify the deposition/extraction event probabilities. Two main questions need explanation: (i) why and whereby which mechanism(s) the tip remains O-terminated after either of the vertical manipulation events? and (ii) why deposition is much more probable than extraction? As it is practically impossible to shed more light on these questions from the experiment alone, we turn to modelling to face these challenges. Modelling: the direct approach When placing a single Cu adatom on the p (2 × 1) reconstructed surface, we find in our DFT simulations that the Cu atom occupies the ‘super’-Cu position, which is very similar to that on the c (6 × 2) surface [12] , [19] (see Fig. 1a and Supplementary Information ). The interaction of the tip [12] (see Fig. 2 ) with a single ‘super’-Cu atom was studied. The energy barrier for taking the ‘super’-Cu atom from the surface to the O-terminated tip between states S and T in Fig. 2 is >1 eV, unless the tip is positioned unreasonably close, <2.0 Å, to the surface. As the experiments were conducted at a temperature of 78 K, the investigated direct transitions would correspond to such negligible rates that can be disregarded altogether. 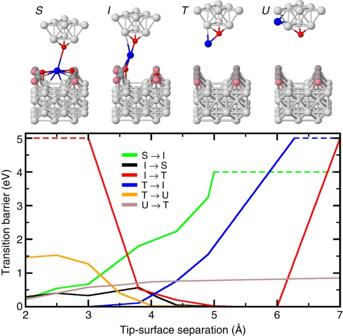Figure 2: The model and computed barriers. Upper panel: The four states of the ‘super’-Cu atom in the surface-tip system:S,I, tipTstate and upper tipUstate; for details, see the text. Colour coding as inFig. 1a. Lower panel: Calculated energy barriers for different transitions betweenS,I,TandUstates of the ‘super’ Cu atom in the surface–tip junction as a function of the tip height. The horizontal dashed lines indicate tip heights at which the transition barrier was assumed constant at the high value indicated; no calculation was performed in this region as the transition probability is too low. Figure 2: The model and computed barriers. Upper panel: The four states of the ‘super’-Cu atom in the surface-tip system: S , I , tip T state and upper tip U state; for details, see the text. Colour coding as in Fig. 1a . Lower panel: Calculated energy barriers for different transitions between S , I , T and U states of the ‘super’ Cu atom in the surface–tip junction as a function of the tip height. The horizontal dashed lines indicate tip heights at which the transition barrier was assumed constant at the high value indicated; no calculation was performed in this region as the transition probability is too low. Full size image Four-state model and energy barriers Next a four-state model taking explicit account of the tip motion was considered (see Fig. 2 ). We found that for tip heights z T ε(2–5) Å from the surface, the Cu atom can be stabilized between its surface state S , and tip state T . This position designated as intermediate state I is shown in Fig. 2 along with the calculated energy barriers Δ E S → I for the S → I transitions at different tip heights z T . One can see that the S → I barrier remains <0.5 eV for the tip heights <≈2.5 Å; further increase of z T results in the barrier increasing dramatically, whereas the barrier for the reverse I → S transition fluctuates around 0.4–0.5 eV and then drops to 0 around z T ≃ 4.5 Å. Once in state I , the Cu atom can be dragged by the tip up to the height of z T ≃ 5.0 Å, where the barrier Δ E I → T for the I → T transition drops to 0 ( Fig. 2 ), or may return back to the surface via equally small Δ E I → S barrier. Once the state T is reached the system spontaneously assumes a new upper tip state U ( Fig. 2 ) as the T state is metastable at large z T (ref. 16 ). To reach this state, the Cu atom diffuses up the tip structure, exposing again the O atom tip termination to the surface. It is essential that the T → U transition only happens after z T ≥4.0 Å, when the corresponding barrier becomes very small (see Fig. 2 ). Once the state U is reached, the Cu atom remains on the tip as the energy barrier to jump back into state T is fairly large ( ≃ 0.8 eV) when the tip is sufficiently far away from the surface [16] . The fact that at some tip heights the Cu atom may jump to the tip and then diffuse up its cone-like structure ( Fig. 1b ) is essential for understanding the experimental observation that the contrast remains the same after a Cu atom is picked up from the surface; this is because the O atom at the tip apex is the closest to the surface before and remains such after the transition, and hence the contrast does not change significantly [16] . The proposed extraction mechanism of vertical manipulation suggests also an explanation for the reverse U → S deposition process via T and I states, see the corresponding reverse barriers in Fig. 2 and Supplementary Information . KMC modelling of tip motion and probabilities To better understand the stochastic nature of the vertical manipulations and work out their probabilities, we have developed a new KMC scheme based on the ideas of time-variable KMC method [15] (see the details in Supplementary Information ) and performed extensive KMC simulations. As an example we consider explicitly the extraction manipulation. In short, first the initial S → I transition is worked out. This gives the oscillation cycle n and the time τ c within the n -th cycle at which state I is formed. The time τ c corresponds to the tip height z T ( τ c )= z 0 + A cos(2 πfτ c ), where z 0 is the tip average position above the surface, A oscillation amplitude and f oscillation frequency. Next a set of subsequent independent calculations of the corresponding conditional probability P I → U ( τ c ) to reach step U provided that system was in state I created at time τ c during the n -th oscillation cycle was run. The final probability of a successful S → U extraction transition is calculated assuming that transition S → I , which is followed by I → U , may happen during any oscillation cycle n and within any time τ c of the n -th cycle. All quantities in the formula above, the probability densities P S → I , P I → U , transition rates r S → I = ν exp(−Δ E S → I / k B T ), and R S =−ln P S → I (1/ f ) can all be fully determined by KMC modelling. For details and for the discussion of the reverse P U → S deposition probability see Supplementary Information . The individual probabilities appearing in equation (1) are shown in Fig. 3 . The probability P S → I ( n ) for the transitions to happen at the n -th cycle falls off exponentially, but a significant number of transitions require ≈10 9 oscillations to occur. The probability density P S → I ( τ c ) has a nearly Gaussian shape centred around the point of the closest approach ( τ c =1/2 f , that is, at the half period). The results corresponding to higher temperatures show that P S → I ( n ) decays much faster with n (not shown) and the probability density P S → I ( τ c ) moves towards the descending part of the cycle (smaller values of τ c ). 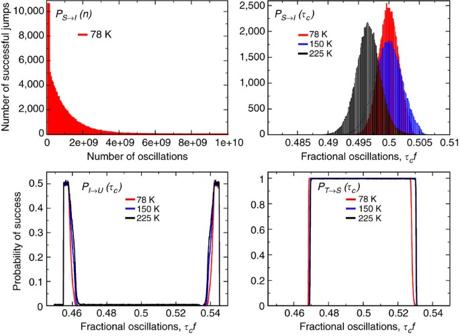Figure 3: KMC results. Upper panel: Calculated statistics for the initialS→Istep of the vertical extraction manipulation with the curves proportional to the probability densitiesPS→I(n) (left) andPS→I(τc) (right). Lower panel: Conditional probability densitiesPI→U(τc) forI→T→Utransition (extraction) andPT→S(τc) for theT→I→Stransition (deposition). Figure 3: KMC results. Upper panel: Calculated statistics for the initial S → I step of the vertical extraction manipulation with the curves proportional to the probability densities P S → I ( n ) (left) and P S → I ( τ c ) (right). Lower panel: Conditional probability densities P I → U ( τ c ) for I → T → U transition (extraction) and P T → S ( τ c ) for the T → I → S transition (deposition). Full size image At all temperatures the conditional probability P I → U ( τ c ) ( Fig. 3 ) is non-zero only within two narrow regions of the tip positions around f τ c ≃ 0.46 (approach) and f τ c ≃ 0.54 (retraction), both corresponding to z T ≃ 5.0 Å. This behaviour can be understood as a result of the competition between I → T and I → S processes, both having very similar transition barriers. In the deposition manipulation the initial stage consists of the U → T transition, which, similarly to extraction, may need many tip oscillations until state T is reached (see Supplementary Information ). However, the conditional probability P T → S ( τ c ) ( Fig. 3 ) shows that in this case the Cu atom prepared in state T anywhere within the time interval f τ c =0.47−0.53 (2.0≤ z T ≤3.5 Å) around the distance of closest approach reaches state S with 100% probability irrespective of temperature. This finding is crucial for understanding the differences between the extraction and deposition manipulations. The calculated final probabilities for the Cu atom extraction are 0.05, 0.07 and 0.09 at 78, 150 and 225 K, respectively, and for deposition 0.98 irrespective of the temperature. The differences in the likelihoods of extraction/deposition can easily be understood in terms of differences in the respective P I → U ( τ c )/ P T → S ( τ c ) conditional probabilities ( Fig. 3 ). Although the extraction probability increases slightly with temperature, we expect low (but non-zero) count in observing the ‘super’-Cu atom extraction and a very high probability of their deposition from the tip when scanning the p (2 × 1) terrace, the fact confirmed by our experimental results. We note that in reality the tip does not continuously oscillate above the given point on the surface, as assumed for computational feasibility here, but moves. We expect that the actual probabilities may be reduced. The simple tip model used in our study may also have some effect on the computed properties [12] , [16] . Nevertheless, keeping in mind the experimental limitations, the computed probabilities do agree with our experimental findings at least qualitatively. We observed multiple vertical NC-AFM manipulation events, both extractions and depositions, of Cu atoms on the p (2 × 1) reconstructed Cu(110):O surface. Intriguingly, we find that in all these events the contrast remained the same and that deposition was much more likely than extraction although systematic experimental statistics is difficult. The fact that our observation is not limited only to the system studied here but is a more general phenomenon is supported by the work of Sugimoto et al. [10] , who observed exchange NC-AFM manipulation without tip modification. However, their observation was limited to one special tip structure occasionally generated in a subset of experiments, which, at variance to our case, neither could be systematically controlled experimentally nor was the mechanism behind that observation explained in ref. 10 theoretically. Using DFT theory in conjunction with KMC simulations, we were able to propose atomic-scale mechanisms for both types of the vertical manipulation, which fully explain our experimental observations. Namely: (i) the tip before and after manipulation remains O-terminated and hence there is no change of imaging contrast since the Cu atom extracted from the surface climbs up the tip structure to occupy a more energetically favourable position; at the same time, the barrier for this atom to leave this state is reduced at close approach to such extent that its deposition becomes very likely; (ii) both manipulations are of inherently stochastic nature, although the extraction transition must be much rarer than the deposition transition. Theory suggests that both transitions consist of a sequence of steps, containing both activation and dragging (no activation required). We find that in this case when trying to work out the underlying atomistic mechanics just an energetic consideration may be misleading and a consideration of kinetics is essential. Our manipulation process belongs to a class characterized by a strong tip-height dependence of energy barriers between the intermediate states encountered, with barrier reduction in some cases with the tip close to and in other cases far away from the surface ( Fig. 2 ). Hence, while the manipulation proceeds easily in the NC-AFM microscope where the tip oscillates, the manipulation would not happen in an apparatus operating in a constant tip–sample distance regime, such as STM. The theory we have developed here is completely general and applicable equally to both vertical and lateral manipulations, which we expect to be required for a full understanding of the majority of NC-AFM/STM manipulations. We expect to find qualitatively similar behaviour, albeit with different states and transition rates, also in manipulation of other systems, such as, for instance, oxidized Cu(100), Ag(100), Ag(110), Ag(111), Ni(110) and Au(110), all of which have either a missing row reconstruction or distinct and different arrangements of metal and oxygen atoms. The metal-oxide surfaces play an important role in their own catalytic reaction [20] , [21] , in serving reaction centres associated with structural defects and adsorbed metal atoms on the surface [22] , [23] and in electronic modification of adsorbed metal atoms [22] , [23] . In fact, the structures formed by our manipulation processes are atomic realizations of dip-pen nano-lithography [10] , [24] , where metal wires are written by the tip on a semiconducting oxide layer grown on metallic copper substrate ( Fig. 1f ). Further development and application of related nano-manipulations could encompass creation of magnetic nanostructures on surfaces with relevance for spintronics [25] and quantum computing [26] , or á la carte creation of active sites on catalyst surfaces. NC-AFM manipulation experiments The experiments were carried out using a home-built NC-AFM operating under ultrahigh vacuum conditions at 78 K. To detect the tip–sample interaction, the frequency-modulation technique was used [27] . Low-resistivity (0.01–0.025 Ω cm) n-doped commercial silicon cantilevers (PPP-NCLR, Nanoworld, Switzerland) were oscillated by keeping the oscillation amplitude constant at A =67 Å. The cantilevers typically had a Q -factor of 150,000, spring constant of 40 N m −1 and resonance frequencies of f =150 kHz. The radius of curvature of the tip apex was <10 nm. The tip is shaped like a polygon-based pyramid with a height of 10–15 μ m. The frequency shift of the oscillating cantilever was measured by using phase-locked-loop-based commercial electronics (easyPLL plus detector and controller, Nanosurf, Switzerland). The Cu(110):O surface was prepared by first cleaning by repeated Ar ion sputtering (1,200 eV) and then annealing at 550 °C, followed by exposure to 2,000 l of oxygen at 300 °C. The tip apex was cleaned by Ar ion sputtering (650 eV) in situ and was found to have a radius of curvature <100 Å. Both the cantilever and the sample were always electrically grounded. Manipulation experiments were performed by scanning a chosen area of the surface with the frequency shift more negative (by −3.5 Hz) compared to the value used for non-intrusive imaging. Simulating energy barriers The surface was modelled using a four-layer slab with the upper two atomic layers allowed to relax [16] , [19] . To model the tip we used a relatively stiff O-terminated Cu tetrahedron [12] , [16] , see also Fig. 2 , with the lowest four atoms allowed to relax upon interaction with the surface. Calculations of the energies and forces were performed using DFT with Perdew–Burke–Ernzerhof density functional [28] and projector augmented-wave pseudopotentials [29] as implemented in the VASP code [30] . Since van der Waals interactions were found to be essential for the O-terminated Cu surfaces [19] , this interaction was accounted for here using the DFT-D2 scheme [31] . Energy barriers were calculated using the Nudged Elastic Band method [32] . The barriers were then used in calculating the corresponding transition rates by employing transition state theory. Modelling of tip dynamics and probabilities Calculations of the dynamics of this system with standard KMC are impossible because while the tip moves the transitions rates strongly depend on time, making the main assumption of the standard KMC theories [33] invalid. The calculation can be done using the fixed time step KMC dynamics method [15] , [34] that was adopted for this study. More details can be found in Supplementary Information . How to cite this article: Bamidele, J. et al. Vertical atomic manipulation with dynamic atomic-force microscopy without tip change via a multi-step mechanism. Nat. Commun. 5:4476 doi: 10.1038/ncomms5476 (2014).